Activating MET kinase rearrangements in melanoma and Spitz tumours Oncogenic gene fusions have been identified in many cancers and many serve as biomarkers or targets for therapy. Here we identify six different melanocytic tumours with genomic rearrangements of MET fusing the kinase domain of MET in-frame to six different N-terminal partners. These tumours lack activating mutations in other established melanoma oncogenes. We functionally characterize two of the identified fusion proteins (TRIM4-MET and ZKSCAN1-MET) and find that they constitutively activate the mitogen-activated protein kinase (MAPK), phosphoinositol-3 kinase (PI3K) and phospholipase C gamma 1 (PLCγ1) pathways. The MET inhibitors cabozantinib (FDA-approved for progressive medullary thyroid cancer) and PF-04217903 block their activity at nanomolar concentrations. MET fusion kinases thus provide a potential therapeutic target for a rare subset of melanoma for which currently no targeted therapeutic options currently exist. Constitutive activation of signalling pathways controlling cell growth and proliferation by activating mutations in dominant oncogenes such BRAF , NRAS , KIT , GNAQ or GNA11 is found in the majority of melanocytic neoplasms [1] , [2] , [3] , [4] , [5] . These mutations tend to occur early during progression and are found in a mutually exclusive pattern in early-stage disease. While inactivating mutations in NF1 have emerged as an additional genetic alteration [6] , a subset of melanomas remains ‘wild-type’ despite exhaustive studies sequencing the coding regions of genes [7] , [8] . Recently, we and others described recurrent rearrangements of kinases as a novel class of oncogenic alterations in this subset of melanocytic neoplasms [9] , [10] , [11] , [12] . In some cases the resulting breakpoints were affected by copy-number changes that increased the gene dosage of the resulting fusion kinases. In our clinical practice, we perform array comparative genomic hybridization (aCGH) as an adjunct to histopathologic diagnosis for difficult to classify melanocytic tumours. In our database of copy-number profiles ( n =1,202), we noticed cases with copy-number transitions within the MET locus on chromosome 7q31.2, resulting in amplification or gain of the 3′ end of the gene that encodes the kinase domain in 7 of 1,202 cases, suggesting the presence of a MET fusion kinase in these cases. MET is the high-affinity tyrosine kinase receptor for hepatocyte growth factor. It functions in angiogenesis, cellular motility, growth and invasion [13] , [14] . In addition, MET plays a role in melanocyte development and homeostasis [15] , [16] , [17] . In 1984, it was identified as a proto-oncogene when TPR-MET, a constitutively active MET fusion kinase, was isolated from a human cell line chemically transformed in vitro [18] ; however, initial reports of TPR-MET expression in human cancer were not replicated [19] , [20] , [21] . MET amplification has been observed in various cancers [22] , [23] , [24] , [25] , [26] and leads to acquired resistance to EGFR inhibitors [27] , [28] , [29] . Recently, alterations within introns of MET that alter protein structure have been identified. Splice site mutations that result in exon 14 skipping, deletion within the juxtamembranous domain of MET, and increased MET activity have been identified in lung adenocarcinomas [30] , [31] . In secondary glioblastomas, fusions within MET intron 1 result in the N terminus of PTPRZ1 fused to the entirety of MET with elevated expression of the MET fusion regulated by the PTPRZ1 promoter [32] . Here we identify gene rearrangements of MET resulting in in-frame MET kinase fusions in Spitz tumours and melanoma. MET fusions appear in a mutually exclusive pattern with previously identified melanoma oncogenes, are constitutively active and tumorigenic, and thus may serve as therapeutic targets for a subset of melanomas. Identification of MET kinase fusions For six of seven cases with copy-number transitions within the MET locus (those from which leftover archival material was available), we performed targeted sequencing of ∼ 300 melanoma and cancer-related genes ( Supplementary Data 1–4 ). Our target regions included MET introns 13–16, which we selected as they are situated upstream of the kinase domain and overlap the areas of copy-number transition we identified in MET . A rearrangement within intron 14 of MET was identified in four of the six tumours ( Figs 1 and 2 , Supplementary Figs 1 and 2 ). In the two tumours without detectable MET fusions, activating BRAF fusions (on chromosome 7q34) were identified instead. The four tumours that harboured MET fusions demonstrated gain of the distal portion of the long arm of chromosome 7. To look for additional cases with MET fusions, we performed targeted sequencing of 41 additional tumours that had copy-number gains of the distal portion of the long arm of chromosome 7 ( Supplementary Fig. 3 , Supplementary Data 5 ). Most of these tumours had copy-number transitions near the MET locus but none had copy-number transitions within MET . However, two of these 41 cases also showed a rearrangement within intron 14 of MET by targeted DNA sequencing. None of the six cases with MET rearrangements had activating mutations in BRAF , NRAS , HRAS , GNAQ , GNA11 or rearrangements of ALK , BRAF , NTRK1 , RET , ROS1 . 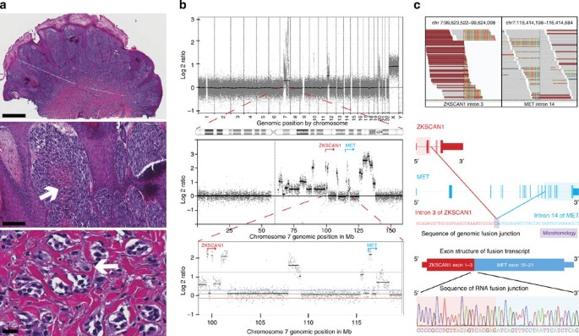Figure 1: Spitzoid melanoma with ZKSCAN1-MET fusion. (a) Histopathology (× 4, scale bar, 1 mm) showing a dome-shaped nodule with a thickened epidermis and sheets of spindled and epithelioid melanocytes in the dermis, some with central necrosis (× 20, arrow, scale bar, 200 μm). High-power view (× 20, lower panel) demonstrates small nests of melanocytes in infiltrative array and a mitotic figure (arrow) in the deep portion of the tumour. Scale bar, 25 μm. (b) aCGH profile (top panel) with copy-number increases involving chromosomes 7 and 12p. Chromosome 7 shows amplification of multiple regions on the long arm, including the 5′ end ofZKSCAN1(red) and the 3′ end ofMET(blue) (lower panels). (c) Stacks of sequencing reads from Integrated Genome Viewer spanning the breakpoints, with unaligned portions (rainbow-coloured) flanking one side of the fusion junction inZKSCAN1(left) andMET(right). Reads whose mate pair maps to the opposite side of the fusion junction are maroon. The DNA sequence of the fusion junction is displayed, with bases that map toZKSCAN1in red, and those that map toMETin blue with their corresponding gene models above. Two bases of microhomology at the fusion junction are displayed in purple. The exonic structure of the predicted fusion transcript is shown with the sequencing trace from RT-PCR confirming its expression beneath. Figure 1: Spitzoid melanoma with ZKSCAN1-MET fusion. ( a ) Histopathology (× 4, scale bar, 1 mm) showing a dome-shaped nodule with a thickened epidermis and sheets of spindled and epithelioid melanocytes in the dermis, some with central necrosis (× 20, arrow, scale bar, 200 μm). High-power view (× 20, lower panel) demonstrates small nests of melanocytes in infiltrative array and a mitotic figure (arrow) in the deep portion of the tumour. Scale bar, 25 μm. ( b ) aCGH profile (top panel) with copy-number increases involving chromosomes 7 and 12p. Chromosome 7 shows amplification of multiple regions on the long arm, including the 5′ end of ZKSCAN1 (red) and the 3′ end of MET (blue) (lower panels). ( c ) Stacks of sequencing reads from Integrated Genome Viewer spanning the breakpoints, with unaligned portions (rainbow-coloured) flanking one side of the fusion junction in ZKSCAN1 (left) and MET (right). Reads whose mate pair maps to the opposite side of the fusion junction are maroon. The DNA sequence of the fusion junction is displayed, with bases that map to ZKSCAN1 in red, and those that map to MET in blue with their corresponding gene models above. Two bases of microhomology at the fusion junction are displayed in purple. The exonic structure of the predicted fusion transcript is shown with the sequencing trace from RT-PCR confirming its expression beneath. 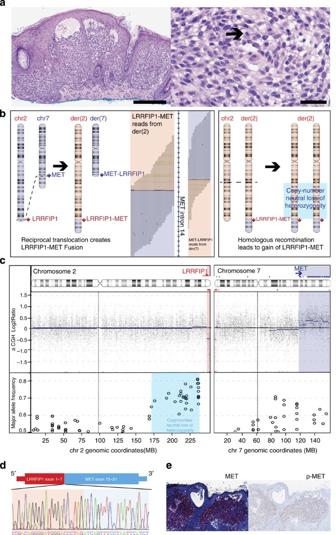Figure 2: Reciprocal translocation resulting in LRRFIP1-MET fusion in an atypical Spitz tumour. (a) Histopathology showing large nests of epithelioid melanocytes with pericellular clefting (× 4, left panel, Scale bar, 300 μm) and scattered mitoses (× 20, right panel, arrow, Scale bar, 50 μm) in the papillary dermis under a thickened epidermis. (b) Inferred succession of genetic events with supporting genomic data. Left panel: reciprocal translocation between chromosomes 2 and 7 generates two derivative chromosomes withLRRFIP1-METandMET-LRRFIP1fusion genes, respectively. Chimeric reads supporting the fusion junctions are mapped to intron 14 ofMETwith the rainbow coloured portion of the reads mapping to chromosome 2. Right panel: subsequent homologous recombination of the derivative chromosome 2 results in a region of copy-number neutral loss of heterozygosity on 2q and gain of theLRRFIP1-METfusion gene. (c) Copy number and major allele frequency plots for chromosomes 2 and 7 demonstrate loss of 2q and gain of 7q distal to the breakpoints and allelic imbalance on 2q. (d) The exonic structure of the predicted fusion transcript with the sequencing trace from RT-PCR confirming its expression. (e) Strong diffuse expression of the kinase domain of MET is demonstrated by immunohistochemistry, with moderate staining for p-MET (× 4, Scale bar, 100 μm). Full size image Figure 2: Reciprocal translocation resulting in LRRFIP1-MET fusion in an atypical Spitz tumour. ( a ) Histopathology showing large nests of epithelioid melanocytes with pericellular clefting (× 4, left panel, Scale bar, 300 μm) and scattered mitoses (× 20, right panel, arrow, Scale bar, 50 μm) in the papillary dermis under a thickened epidermis. ( b ) Inferred succession of genetic events with supporting genomic data. Left panel: reciprocal translocation between chromosomes 2 and 7 generates two derivative chromosomes with LRRFIP1-MET and MET-LRRFIP1 fusion genes, respectively. Chimeric reads supporting the fusion junctions are mapped to intron 14 of MET with the rainbow coloured portion of the reads mapping to chromosome 2. Right panel: subsequent homologous recombination of the derivative chromosome 2 results in a region of copy-number neutral loss of heterozygosity on 2q and gain of the LRRFIP1-MET fusion gene. ( c ) Copy number and major allele frequency plots for chromosomes 2 and 7 demonstrate loss of 2q and gain of 7q distal to the breakpoints and allelic imbalance on 2q. ( d ) The exonic structure of the predicted fusion transcript with the sequencing trace from RT-PCR confirming its expression. ( e ) Strong diffuse expression of the kinase domain of MET is demonstrated by immunohistochemistry, with moderate staining for p-MET (× 4, Scale bar, 100 μm). Full size image In five of six cases (all except case 4), an in-frame fusion transcript containing MET exons 15–21 was predicted based on the DNA sequence. Out of these five cases, four had tissue available for reverse transcription polymerase chain reaction (RT-PCR), which confirmed the presence of the predicted chimeric transcripts in all cases. In case 4, no 5′ partner was identified, as the DNA sequencing data indicated that the 3′ portion of MET starting from within intron 14 of MET was fused to an intergenic region on 7q22.3. Kinome transcriptome sequencing of this case identified in-frame TRIM4-MET fusion transcripts joining exon 6 of TRIM4 to exon 15 of MET and we verified this fusion by RT-PCR. Re-examination of the aCGH profile revealed copy-number gains with similar amplitudes of the 5′ end of TRIM4 , the intergenic region on 7q22.3 fused to MET , and the 3′ end of MET ( Supplementary Fig. 2 ). Altogether, this indicates a complex rearrangement joining intron 6 of TRIM4 to a small intergenic region on 7q22.3 and then on to intron 14 of MET with subsequent copy-number increase of the MET fusion kinase. In case six, two separate breakpoints were identified within MET resulting in four detectable fusion junctions between chromosomes 1 and 7 (with only one fusion junction resulting in a predicted in-frame transcript). The aCGH profile demonstrated alternating copy number of the affected portions of chromosomes 1 and 7, raising the possibility that the MET fusion was the result of chromothripsis ( Supplementary Fig. 4 ). Thus, in two of six cases with MET fusions, we observed evidence of a complex genomic rearrangement that generated the fusions. In cases three and five, we observed reciprocal fusion junctions within 400 base pairs, indicating that the MET fusion resulted from a reciprocal translocation event ( Fig. 2 , Supplementary Fig. 5 ). In case three, the copy-number profile indicated that reciprocal translocation was followed by a homologous recombination event on the larger derivative chromosome, resulting in loss of heterozygosity of a segment from chromosome 2 and copy-number increase of the fusion kinase gene ( Fig. 2b,c ). Gain of the MET fusion gene was observed in three cases and amplification (log2ratio>2) was observed in one case ( Table 1 ), suggesting additional selection for increased dosage of the MET fusion gene during tumour progression. As expression of the MET fusion gene is driven by the promoter of the 5′ partner gene, expression levels should not be related to the basal level of MET expression. In addition, regulation directed at the MET promoter should not affect expression of the MET fusion. It is expected that the normal expression level of the 5′ partner genes in melanocytes determines whether subsequent copy-number gain of the MET fusion gene constitutes a significant fitness advantage. Table 1 Clinical and genetic features of melanocytic tumours with MET fusion kinase. Full size table In all six cases, the neoplastic melanocytes demonstrated a predominance of fusiform and/or epithelioid morphology with moderate to large amounts of amphophilic cytoplasm. These cytologic features are defining characteristics of Spitz tumours [33] . Four of six cases also demonstrated epidermal hyperplasia and large junctional nests of melanocytes, additional features often seen in Spitz tumours, while Kamino bodies (eosinophilic acellular material at the dermo-epidermal junction) and single melanocytes in the upper levels of the epidermis were not observed. We performed MET immunohistochemistry using the three tumours for which material was available. All three cases demonstrated strong diffuse cytoplasmic expression of the kinase domain of MET in neoplastic melanocytes in contrast to common melanocytic naevus control tissue, which showed little or no expression of MET ( Fig. 2e , Supplementary Figs 2d, 4e, 6 ). While not specific for the MET fusion kinase, these results demonstrate increased expression levels of the kinase domain of MET in tumours with MET fusions compared with common nevi. Immunohistochemistry for p-MET (tyrosine 1234/5) demonstrated increased levels of p-MET compared with common melanocytic naevus control tissue ( Fig. 2 , Supplementary Figs 1, 4, 6 ). In all cases, the breakpoint in MET occurred within intron 14 upstream of exons 15–21 of MET , which encode the entire kinase domain of MET ( Fig. 3 ). Exon 14, which encodes the N-terminal portion of the auto-inhibitory juxtamembrane domain and the Cbl binding site Y1003 (important for ubiquitinization, degradation and downregulation of MET), is notably absent in the MET fusions [34] . The diversity of 5′ partners of MET fusions is similar to the diversity of 5′ partners we observed previously for BRAF and ROS1 fusions in Spitz tumours [10] , [12] . Some of the 5′ fusion partners overlap with those previously described: the N-terminus of DCTN1 had been found fused to the kinase domain of ALK and the N-terminus of PPFIBP1 to the kinase domain of ROS1 in Spitz tumours [12] . Similar to the fusion partners of these kinases, the N-terminal fusion partners of MET also contributed multimerization domains, which in five cases were coiled-coil domains and in one case was a SCAN domain ( Fig. 3 ). The finding of an intact MET kinase domain fused to a range of 5′ partner genes involved in other oncogenic kinase fusions and/or with multimerization domains suggests that MET fusions are constitutively active. 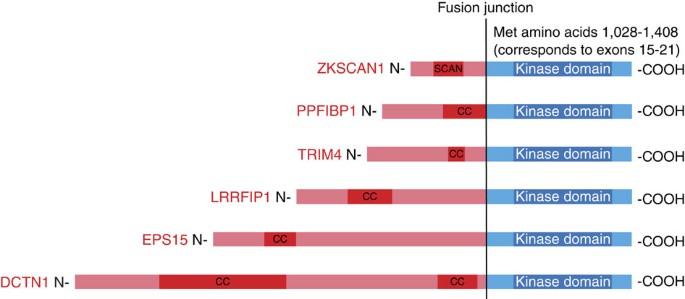Figure 3: Domain structure of MET Fusions. The portion from the N-terminal partner is displayed in pink with multimerization domains highlighted in red (CC=coiled coil domain, SCAN=SCAN domain). The MET portion (starting from exon 15 in all cases) is coloured blue with the kinase domain highlighted in dark blue. Figure 3: Domain structure of MET Fusions. The portion from the N-terminal partner is displayed in pink with multimerization domains highlighted in red (CC=coiled coil domain, SCAN=SCAN domain). The MET portion (starting from exon 15 in all cases) is coloured blue with the kinase domain highlighted in dark blue. Full size image Functional validation To assess this directly, we expressed TRIM4-MET and ZKSCAN1-MET fusion constructs (developed using synthesized theoretical fusion cDNA sequences) in 293FT cells and immortalized mouse melanocytes [35] and found that both fusion kinases were phosphorylated at tyrosine 1234/5 (a marker of kinase activation) under serum-starved conditions with activation of downstream signalling pathways ( Fig. 4a , Supplementary Fig 7 ). In immortalized mouse melanocytes stably transduced with TRIM4-MET or ZKSCAN1-MET , no increase in p-MET, p-ERK, p-AKT or p-PLCγ1 was observed after HGF stimulation in contrast to untransduced melanocytes and melanocytes transduced with wild-type MET ( Fig. 4a ). Insensitivity of the MET fusions to HGF was expected as the extracellular and transmembrane portions of MET are not present and MET fusion kinases are no longer localized to the plasma membrane as supported by cytoplasmic staining by MET and p-MET immunohistochemistry. The absence of wild-type p-MET after HGF stimulation in melanocytes stably expressing MET fusions suggests downregulation of the endogenous wild-type receptor as a cellular response to constitutive signalling of the fusion kinases. Treatment with 100 nM of cabozantinib (a potent but non-specific MET inhibitor, US Food and Drug Administration (FDA) and European Medicines Agency (EMA) approved for progressive medullary thyroid cancer [36] ) or PF-04217903 (a selective MET inhibitor [37] ) for 4 h resulted in decreased p-MET, p-ERK, p-AKT and p-PLCγ1 in melanocytes expressing TRIM4-MET or ZKSCAN1-MET ( Fig. 4b ), demonstrating that both drugs inhibit signalling of MET fusion kinases. 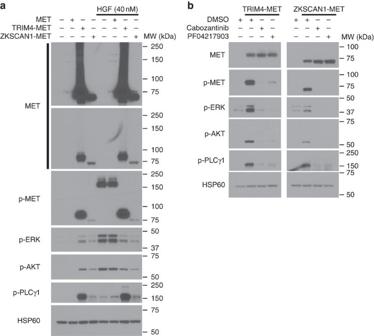Figure 4: MET fusions constitutively activate oncogenic signalling pathways and are inhibited by cabozantinib and PF-04217903. (a) Melan-a cells (immortalized mouse melanocytes) were stably transduced with full-lengthMET, TRIM4-METandZKSCAN1-METexpression constructs. The expressed fusion proteins were detected with by an MET antibody at the predicted molecular weights of 79 and 65 kDa (longer exposure upper MET panel, shorter exposure lower MET panel). TRIM4-MET and ZKSCAN1-MET were phosphorylated at tyrosine 1,234/1,235 in the absence of serum. (b) Treatment with cabozantinib or PF-04217903 for 4 h (both at 100 nM) significantly decreased p-MET and downstream signalling. Figure 4: MET fusions constitutively activate oncogenic signalling pathways and are inhibited by cabozantinib and PF-04217903. ( a ) Melan-a cells (immortalized mouse melanocytes) were stably transduced with full-length MET, TRIM4-MET and ZKSCAN1-MET expression constructs. The expressed fusion proteins were detected with by an MET antibody at the predicted molecular weights of 79 and 65 kDa (longer exposure upper MET panel, shorter exposure lower MET panel). TRIM4-MET and ZKSCAN1-MET were phosphorylated at tyrosine 1,234/1,235 in the absence of serum. ( b ) Treatment with cabozantinib or PF-04217903 for 4 h (both at 100 nM) significantly decreased p-MET and downstream signalling. Full size image Immortalized mouse melanocytes stably transduced with ZKSCAN1-MET formed tumours ( n =6 of 6) within 5 weeks of subcutaneous injection into immunocompromised mice, whereas green fluorescent protein (GFP) expressing control cells ( n =6) formed no tumours after 12 weeks ( Fig. 5 ), demonstrating that ZKSCAN1-MET is tumorigenic. 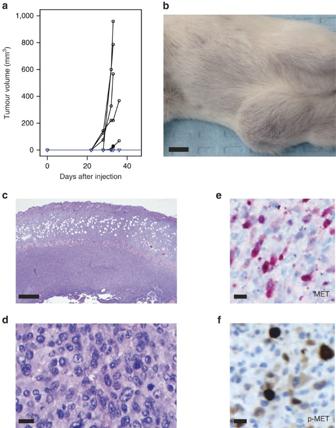Figure 5: ZKSCAN-1 MET is tumorigenic. (a) Melan-a stably transduced with aZKSCAN1-METexpression construct were injected into NOD/SCID/interleukin 2 receptor γ null mice (1.5 million cells, bilateral flank injections) with matched GFP-transduced controls. All six injection sites with ZKSCAN1-MET expressing melan-a cells developed tumours within 5 weeks (black circles), whereas no tumours developed at the sites injected withGFP-transduced controls (n=6) after 12 weeks (blue triangles). (b) Tumour formation 28 days after injection with ZKSCAN1-MET expressing melan-a cells. Scale bar, 0.5 cm. (c) Histopathology of ZKSCAN1-MET tumour (× 4) demonstrates tumour cells diffusely within the skin and subcutaneous tissue. Scale bar, 500 μm. (d) At high power (× 20) tumour cells have hyperchromatic and irregularly sized nuclei and mitoses are present. Scale bar, 10 μm. (e) Tumour cells have variable positivity for the kinase domain of MET (× 20). Scale bar, 10 μm. (f) Tumour cells have variable levels of p-MET positivity (× 20). Scale bar, 10 μm. Figure 5: ZKSCAN-1 MET is tumorigenic. ( a ) Melan-a stably transduced with a ZKSCAN1-MET expression construct were injected into NOD/SCID/interleukin 2 receptor γ null mice (1.5 million cells, bilateral flank injections) with matched GFP-transduced controls. All six injection sites with ZKSCAN1-MET expressing melan-a cells developed tumours within 5 weeks (black circles), whereas no tumours developed at the sites injected with GFP -transduced controls ( n =6) after 12 weeks (blue triangles). ( b ) Tumour formation 28 days after injection with ZKSCAN1-MET expressing melan-a cells. Scale bar, 0.5 cm. ( c ) Histopathology of ZKSCAN1-MET tumour (× 4) demonstrates tumour cells diffusely within the skin and subcutaneous tissue. Scale bar, 500 μm. ( d ) At high power (× 20) tumour cells have hyperchromatic and irregularly sized nuclei and mitoses are present. Scale bar, 10 μm. ( e ) Tumour cells have variable positivity for the kinase domain of MET (× 20). Scale bar, 10 μm. ( f ) Tumour cells have variable levels of p-MET positivity (× 20). Scale bar, 10 μm. Full size image We identified MET fusion kinases in 0.5% of our cohort of 1,202 diagnostically challenging melanocytic tumours by sequencing cases selected for copy-number transitions within MET ( n =6) or copy-number gain of the distal portion of the long arm of chromosome 7 ( n =41). Our approach likely underestimates the frequency of MET fusions in our cohort as such fusions can arise from copy-number neutral structural rearrangements. All cases with MET fusions displayed spitzoid histopathologic features and were diagnosed as Spitz tumours or spitzoid melanoma. Spitz tumour refers to a spectrum of tumours, ranging from benign to malignant that includes Spitz naevus (benign), atypical Spitz tumour (ambiguous biologic potential) and spitzoid melanoma (malignant). They are characterized by spindled or epithelioid melanocytes, more commonly arise in children or young adults and have a lower incidence than nevi and melanomas that do not display these cytologic features [33] . Spitz tumours pose unique diagnostic challenges as their histopathologic features are diverse and often overlap with those of BRAF and NRAS mutant melanoma. Classification of Spitz tumours along the spectrum of benign to malignant shows poor inter-observer reproducibility and poor correlation with clinical outcomes [38] . This may be due to the increased diversity of oncogenic drivers in Spitz tumours as compared with other melanocytic tumours [33] . The tumours with MET fusions occurred in young patients (9–29 years old, average 20 years) similar to what we observed in cohorts of melanocytic tumours with other kinase fusions [10] , [12] . While our cohort of aCGH characterized tumours spans the spectrum of ambiguous melanocytic tumours and includes cases with a possible diagnosis of blue nevus, deep penetrating nevus, ancient nevus, conventional nevus or dysplastic nevus, the majority of cases are Spitz tumours occurring in young patients ( Supplementary Table 1 ). We speculate that MET fusions are associated with spitzoid histopathologic features and are more frequent in younger patients, though this remains to be determined. In other solid tumours such as lung cancer, breast carcinoma and pancreatic carcinoma, variants enriched for activating kinase fusions occur in younger patients [39] , [40] , [41] . The frequency and age distribution of activating MET fusions in melanoma remains to be determined. Analysis of RNA-seq data from nearly 7,700 cancer samples in The Cancer Genome Atlas (TCGA) by Stransky and colleagues identified six MET fusions in thyroid carcinoma, lung adenocarcinoma, papillary renal carcinoma, low-grade glioma and hepatocellular carcinoma, but not in cutaneous melanoma cases ( n =374), indicating that MET fusions are rare in cutaneous melanoma [42] . In two of the six MET fusions in the TCGA, the MET portion of the fusion transcript began with exon 15, similar to the fusions we identified in melanocytic neoplasms. We did not observe copy-number transitions resulting in relative gain of the 3′ end of MET in the TCGA melanoma cases analysed by Stransky et al . (aCGH data available for 373 cases). Notably, the median age of TCGA melanoma patients analysed in this cohort was 56 years with only one patient less than 18 years old (clinical data available for 362 cases). Our finding of MET fusions in tumours that ranged in classification from likely benign to unequivocally malignant indicates that MET fusion kinases occur early during progression. While MET fusions appear rare in melanoma, they lead to constitutively active kinases that can be inhibited by approved drugs. As they occur in a mutually exclusive pattern with activating mutations in known melanoma oncogenes they are likely to represent a therapeutic target in a small subset of melanomas. Study population We analysed a database of 1,202 melanocytic neoplasms, for which aCGH was performed as part of the diagnostic assessment at the Dermatopathology Section of the Departments of Dermatology and Pathology at the University of California, San Francisco over a 36-month period from 2010 through 2013. The majority of these cases are borderline lesions with histopathological features that overlap those of benign nevus and melanoma, for which aCGH was performed as an ancillary diagnostic test. The final diagnosis was determined by review of the final pathology report for each patient. The morphologic classification of the tumour types into Spitz, conventional, deep penetrating nevus-like, or blue nevus-like was determined by review of the final pathology reports and the microscopic descriptions. The study was approved by the Committee on Human Research and was conducted according to the Declaration of Helsinki. Human tissues were obtained with informed consent during the course of clinical care and a waiver of consent was granted for use of archival material in this study. DNA and RNA extraction Areas of tumour were microdissected from 20-μm sections of formalin-fixed, paraffin-embedded (FFPE) tumour. After deparaffinization by washing with Safeclear and ethanol, DNA was extracted by phenol chloroform extraction. RNA was extracted from FFPE tumour after microdissection using the Qiagen RNEasy FFPE kit (p/n 73504) following the manufacturer’s protocol. Array comparative genomic hybridization aCGH was carried out with 500–1,000 ng of genomic DNA on Agilent 4 × 180 k microarrays (Agilent, Santa Clara, CA). The raw microarray images were processed with Agilent Feature Extraction software and analyzed using Nexus Copy Number Software version 7.0 (Biodiscovery, El Segundo, CA). Cases demonstrating copy-number transitions with copy-number increase of the 3′ portion of MET and with sufficient residual DNA or tissue were selected for sequencing. A total of 74 cases were identified with gain of the distal portion of the long arm of chromosome 7 (including the six cases with MET copy number transitions). Of the 68 cases without copy-number transitions in MET , 41 with sufficient residual DNA or tissue were selected for sequencing. DNA sequencing and analysis Multiplex library preparation was performed using the Ovation Ultralow Library System (NuGEN, San Carlos, CA, p/n 0331-32) or NEXT flex Pre-Capture Combo DNA Library Prep Kit (Bioo Scientific, Austin, TX, p/n No. 5140-53) according to the manufacturer’s specifications with 200 ng of sample DNA. Hybridization-capture of pooled libraries was performed using custom-designed bait libraries (Nimblegen SeqCap EZ Choice, p/n 06588786001) spanning ∼ 1.8 Mb of the genome including the exons of BRAF , NRAS , HRAS , KIT , GNAQ and introns 13–16 of MET ( Supplementary Data 1–4 ). The target intervals cover mostly exonic but also some intronic and untranslated regions of 293 (version 1) or 365 target genes (version 2). The target genes were curated to comprise common cancer genes with particular relevance to melanoma. Captured libraries were sequenced as paired-end 100 bp reads on a HiSeq-2000 or HiSeq2500 instrument (Illumina). Sequence reads were mapped to the reference human genome (hg19) using the Burrows-Wheeler aligner (BWA) [43] . Recalibration of reads and variant calling were performed using the Genome Analysis Toolkit (GATK) [44] . Coverage and sequencing statistics were determined using Picard CalculateHsMetrics and Picard CollectInsertSizeMetrics. Variant annotation was performed with Annovar [45] . For fusion detection, read pairs with one or more reads unaligned, insert sizes >1,000 bp, or with soft clipping of at least one read were extracted and re-aligned using BWA-SW [46] and used as input to CREST [47] . Structural variants predicted by CREST were reviewed by visual inspection in the Integrative Genomics Viewer [48] . We predicted the resulting fusion transcripts by joining the exon directly upstream from the genomic breakpoint with the exon directly downstream. Predicted protein sequences were then determined from the predicted transcripts. RNA sequencing and analysis Double-stranded cDNA was synthesized with the NEBNext mRNA Library Prep Reagent Set for Illumina (New England Biolabs E6100S) with 250 ng of input total RNA. Hybrid selection of indexed, adaptor-ligated libraries was performed using the cDNA Kinome hybridization kit with 612 transcripts of kinases and kinase-related genes (Agilent SureSelect Human Kinome Kit, 5,190-4,801). Sequencing was performed on the HiSeq-2500 instrument (Illumina) with paired-end 100 bp reads. Sequence reads were mapped to the reference human genome (hg19) using Spliced Transcripts Alignment to a Reference (STAR) [49] . Confirmation by RT-PCR Total RNA extracted from FFPE tissue sections was reverse transcribed with random hexamer primers using the NEBNext RNA First Strand Synthesis module. PCR to detect the fusion identified by genomic sequencing was performed with negative controls ( Supplementary Table 2 ). The transcript fusion sequence was confirmed by Sanger sequencing (Quintara Biosciences). Plasmid construction The cDNA of the TRIM4-MET and ZKSCAN1-MET fusions were directly synthesized (GENEWIZ) and subsequently cloned into pENTR with the D-TOPO cloning kit as per manufacturers instructions. Subsequently, the cDNAs were cloned by LR Clonase II (Life Technologies) into the pLenti6.3/TO/V5-Dest backbone (Life Technologies). Generation of stably transduced cell lines Melan-a cells were generously provided by Dr Dorothy C. Bennett (St George’s Hospital, University of London, London, UK) [50] and maintained in glutamine-containing RPMI-1640 supplemented with 10% heat-inactivated fetal bovine serum, 200 nM of 12-O-tetradecanoylphorbol-13-acetate (TPA), penicillin (100 units ml −1 ) and streptomycin (50 mg ml −1 ). 293FT cells were purchased from Life Technologies and maintained in DME-H21 medium containing 10% heat-inactivated fetal bovine serum, minimal essential media (MEM) non-essential amino acids (0.1 mM), sodium pyruvate (1 mM), penicillin (100 units ml −1 ) and streptomycin (50 mg ml −1 ). Lentiviruses were produced by transfecting 293FT cells with plasmid DNA (pLenti6.2-GFP, pLenti6.3/TO/V5-Dest-TRIM4-MET, or pLenti6.3/TO/V5-Dest-ZKSCAN1-MET with pCMV-VSV-G and pCMV delta R8.2 using Lipofectamine 2000 (Life Technologies). Stably transduced melan-a cells expressing TRIM4-MET or ZKSCAN1-MET were generated by infection with lentivirus in the presence of 10 μg ml −1 of polybrene (Santa Cruz Biotechnology). Cells were selected for at least 20 days using 5 μg ml −1 of blasticidin S-hydrochloride (Life Technologies) after lentiviral infection. Drug studies The FDA-approved MET inhibitor cabozantinib [51] and more selective MET inhibitor PF04217903 [37] were purchased from Selleckchem (Houston, TX). Stably transduced melan-a cells were treated with glutamine-containing RPMI-1640 with and without drug (100 nM) for 4 h before collection of lysates. Western blotting Antibodies: anti-phospho-Erk (#9101), anti-Met (#8198), anti-phospho-Met (Tyr1234/1235) (#3077), anti-phospho-PLCγ1 (Tyr783) (#2821), from Cell Signaling Technologies, anti-HSP60 (sc-1722) from Santa Cruz Biotechnology. Cell lysates were prepared in RIPA buffer supplemented with Halt protease and phosphatase inhibitor cocktail (Thermo Scientific). Equal amounts of protein, as measured by bicinchoninic (BCA) protein assay, were resolved in 4–12% Bis-Tris NuPage gradient gels (Life Technologies) and transferred electrophoretically to a polyvinylidene difluoride 0.45 μM membrane. Membranes were blocked in 5% non-fat milk in Tris-buffered saline and Tween 20 (TBST) before being incubated overnight at 4 °C with the primary antibodies (1:1,000 dilution in 5% non-fat milk in TBST). Signal detection was achieved by incubation of the membrane in enhanced chemiluminiscent (ECL) solution (Millipore) and autoradiography film exposure. The full blots are shown in Supplementary Figs 8 and 9 . Tumorigenicity study Animal experiments were carried out in accordance with the Declaration of Helsinki and were approved by the ethical committee of the University of California, San Francisco. Bilateral injections of 1.5 million melan-a cells stably transduced with the ZKSCAN1-MET fusion or a GFP control vector were performed on 6-week-old female non-obese diabetic/severe combined immunodeficiency, interleukin-2-Rγ null mice. Detection of tumour was performed by palpation three times a week and tumour volumes were calculated using the formula V =( L × W 2 )/2 over a period of 12 weeks or until the animal had to be killed. Accession codes: The RNA and DNA sequence data have been deposited in the GenBank sequence read archive (SRA) under the accession code SRP033273 . The aCGH data have been deposited in the Gene Expression Omnibus database under accession code GSE67841 . How to cite this article: Yeh, I. et al . Activating MET kinase rearrangements in melanoma and spitz tumours. Nat. Commun. 6:7174 doi: 10.1038/ncomms8174 (2015).